Experimental demonstration of low-loss optical waveguiding at deep sub-wavelength scales Emerging communication applications call for a road map towards nanoscale photonic components and systems. Although metal-based nanostructures theoretically offer a solution to enable nanoscale photonics, the key demonstration of optical modes with deep sub-diffraction-limited confinement and significant propagation distances has not been experimentally achieved because of the trade-off between optical confinement and metallic losses. Here we report the first experimental demonstration of truly nanoscale guided waves in a metal– insulator–semiconductor device featuring low-loss and broadband operation. Near-field scanning optical microscopy reveals mode sizes down to 50×60 nm 2 at visible and near-infrared wavelengths propagating more than 20 times the vacuum wavelength. Interference spectroscopy confirms that the optical mode hybridization between a surface plasmon and a dielectric mode concentrates the hybridized mode inside a nanometre thin gap. This nanoscale waveguide holds promise for next generation on-chip optical communication systems that integrate light sources, modulators or switches, nonlinear and quantum optics. Photonics has become the key driver in global data communications. The ever growing demand for higher data bandwidth and lower power consumption of photonic devices [1] , [2] has set a roadmap for reducing the physical photonic component size down to the nanoscale beyond the diffraction limit of light, with integrated functionality [2] , [3] , [4] , [5] . Although various compact technologies have been developed for reducing the physical size of devices [1] , [4] , [5] , strong optical mode confinement offers enhanced light-matter interactions [6] , [7] , [8] , [9] , [10] , [11] , [12] , [13] , [14] towards low driving power and fast modulation speeds [15] , [16] , [17] , [18] , [19] , [20] . Optical confinement in conventional photonic components is restricted by the diffraction limit of the light resulting in weak light-matter interaction that often demands long device sizes to achieve an effect. For example, ring resonators [4] and Fabry–Perots [20] often require large cavity lengths of 10–1,000 μm leading to relatively large footprints, thermal instabilities [5] and high bending-induced radiation losses on downscaling ring resonators [21] . Surface plasmon polaritons [6] , collective oscillations of electrons at metal-dielectric interfaces, were proposed as a potential solution for nanoscale photonics as their wavelength can be scaled down below diffraction limit [6] , [7] , [8] , [22] . However, the direct experimental demonstration of low-loss propagation of deep sub-wavelength optical modes has not been realized because of the rapid increase in the optical mode's propagation loss on scaling down the optical mode, which pushes the electromagnetic field into the metal [8] , [9] , [10] , [22] , [23] , [24] , [25] . As a result, the use of plasmonics for integrated photonics, in particular for optical interconnects, remains uncertain. A hybrid plasmon polariton (HPP) concept has been proposed to overcome this challenge [11] , [26] , [27] . This approach uses a high dielectric constant semiconductor strip separated from a metal surface by a nanoscale low dielectric constant gap. As the hybridized plasmon energy is concentrated in the low-loss gap, this novel method offers ultra-small mode confinement ( λ 2 /400) over a broad range of frequencies and simultaneously allows for reduced optical loss compared with a metal–semiconductor interface design [11] , [12] . The physical origin of this quasi-TM highly confined mode stems from the continuity requirement of the vertical component of electric displacement ( D y ) at the high-index contrast interfaces between the high-index material (for example, semiconductor), the low-index gap region and plasmonic metal. Experimental design to probe sub-wavelength mode By utilizing semiconductor and metallic structures in an integrated design, in this paper, we report the first observation of long-propagating optical waveguiding revealing mode sizes significantly below the diffraction limit of light visualized by apertureless near-field scanning optical microscopy (NSOM; Fig. 1a; Methods and Supplementary Fig. S1a ). Moreover, unlike other non-resonant plasmonic designs [9] , [10] , [22] , [23] , [24] , [25] , this HPP concept features both ultra strong optical confinement over a broad wavelength range ( λ =633 nm–1.43 μm) and relatively low metal losses with propagation distances exceeding 20 times its free-space wavelength at near infrared, making it a promising candidate for nanophotonics [2] . The measured optical mode sizes down to 53×63 nm 2 are in excellent agreement with theoretical simulations. To visualize the extremely small scales of the HPP mode distribution, we fabricated HPP-based strips with lateral dimensions of about 200 nm in height, H , with varying width, W (150–800 nm). 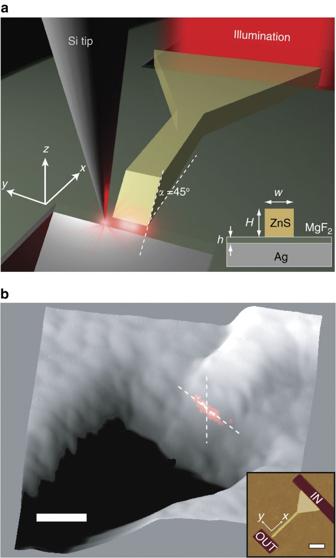Figure 1: HPP mode mapping using near-field scanning optical microscopy (NSOM). (a) Schematic of HPP mode size mapping via apertureless NSOM. The HPP strips consist of a semiconductor strip separated from a metallic surface by a nanometre-scale low dielectric constant gap and are excited by illuminating a metal slit at the input end. (b) Three-dimentional image overlap of the deep sub-wavelength HPP mode signal (red spot) offering optical confinement significantly below the diffraction limit of light. This degree of optical confinement indicates the devices' potential to create strong light-matter interaction for compact and highly functional photonic components. Scale bar, 125 nm. MgF2gaph=10 nm, illumination wavelengthλ=633 nm. Inset: height profile of tapered strip for free space to HPP strip coupling, scale bar, 1 μm. Focused ion beam (FIB) etching was used to define the illumination port (IN) and the access point for the NSOM probe of the confined optical mode (OUT) (seeMethodsfor fabrication details). Figure 1b shows a topological atomic force microscopy scan with the shown region being close to the diffraction limit of light around the output of such a strip superimposed with the NSOM image acquired simultaneously at an illumination wavelength of 633 nm. It can be seen that the optical confinement is indeed as small as about 50 nm (full-width at half-maximum, FWHM) and is situated at the dielectric constant gap region directly confirming the HPP mode. Figure 1: HPP mode mapping using near-field scanning optical microscopy (NSOM). ( a ) Schematic of HPP mode size mapping via apertureless NSOM. The HPP strips consist of a semiconductor strip separated from a metallic surface by a nanometre-scale low dielectric constant gap and are excited by illuminating a metal slit at the input end. ( b ) Three-dimentional image overlap of the deep sub-wavelength HPP mode signal (red spot) offering optical confinement significantly below the diffraction limit of light. This degree of optical confinement indicates the devices' potential to create strong light-matter interaction for compact and highly functional photonic components. Scale bar, 125 nm. MgF 2 gap h =10 nm, illumination wavelength λ =633 nm. Inset: height profile of tapered strip for free space to HPP strip coupling, scale bar, 1 μm. Focused ion beam (FIB) etching was used to define the illumination port (IN) and the access point for the NSOM probe of the confined optical mode (OUT) (see Methods for fabrication details). Full size image The HPP strips are excited by illuminating a metal slit at the input (IN) end of the strip (inset of Fig. 1b ) from the substrate side with polarization perpendicular to the slit. As our near-field imaging technique is most sensitive to electric fields along the axis of the NSOM detection tip, the z -component of the HPP mode is imaged, which is expected to be strongest in the gap region. To gain access to the internal fields, we sliced the strip open ( Fig. 1b ) allowing the NSOM tip to probe the HPP mode's cross-section directly (Methods). When the polarization of illumination is parallel to the metal slit, HPP modes are not excited in the strip and only a background signal was measured by the NSOM (see Supplementary Material ). Broadband HPP mode mapping for height and width We have compared line-scans of the NSOM field image (broken white lines in Fig. 1b ) with numerical simulations. Taking into account the HPP mode's field diffraction along the z -direction, we were able to correlate experiment and theory well at tip-sample separations of about 10 nm ( Fig. 2a ). A similar correlation is found for the mode width data along the y -direction. The optical mode confinement in the y -direction is controllable by the lateral HPP strip width, W , with the smallest measured mode area, A HPP =53×63 nm 2 , proving a non-resonant, deep sub-wavelength (< λ /10, λ =633 nm) nanoscale mode. 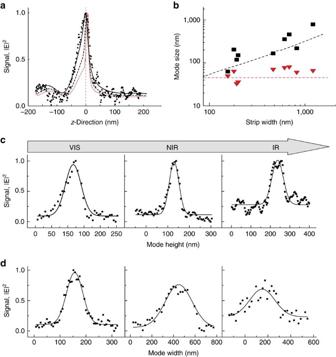Figure 2: HPP mode confinement. (a) Experimental field intensity (black dots) of the HPP mode compared with different tip-sample separations,t, from its exiting point. The optical mode height of FWHMz=53 nm is deep sub-wavelength forλ=633 nm, HPP strip dimensionsH=230 nm,W=174 nm. Note, the NSOM operates in tapping-mode having an average separation oft=10 nm (black line), and the simulated mode profile (t=2 and 5 nm, red dotted and black dashed line, respectively) at this distance agrees well with the NSOM result. (b) Summary of experimental HPP mode dimensions yielding the smallest measured mode area of 53×63 nm2, atλ=633 nm. The good agreement between experimental data (mode width and height, black squares and red triangles, respectively) and theoretical simulations (dashed lines, colours, respectively) confirms that the optical HPP mode is indeed squeezed into the low dielectric constant gap: the mode height is independent on the strip width (triangles), whereas the mode width is scaling with the strip width (squares). (c,d) Line scans of the mode height and width for wavelengths of the illumination beam of 633, 808 and 1,427 nm featuring broadband, deep sub-wavelength operation of HPP-based devices. The FWHM (solid line) are Gaussian fits to binned data, yielding measured mode areas ofλ2/120,λ2/59 andλ2/157, which are deep sub-wavelength modes for all three wavelengths. As the strip height,H, is optimized for 633 nm, a slightly larger mode height for longer excitation wavelengths is expected. Figure 2b summarizes this property by comparing the FWHM of the HPP mode for varying HPP strip widths. Whereas the mode height in the z -direction remains essentially constant, the mode width follows the strip width. Whereas deep sub-wavelength mode sizes are expected in the z -direction because of the involvement of surface plasmons, lateral confinement can also be strongly sub-wavelength. This arises from the accumulation of polarization surface charges concentrated around the centre ( y -direction) of the HPP strip [11] ( Supplementary Fig. S2 ). We have chosen to use FWHM as a measure of the mode size, as it is representative of where the majority of a mode's power resides. This is particularly relevant to active applications of plasmonics, where interest resolves around achieving high peak field intensities within waveguides. We note that this measure can underestimate the mode size in some plasmonic waveguide systems that involve sharp metal corners or large changes in permittivity [12] . However, in our experiments, diffraction of the confined mode into free space and the point spread function of the NSOM tip smooth out the mode's sharp features making the FWHM a fair representation of where the majority of the mode's power resides. Furthermore, we find the hybrid plasmon mode's confinement to be relatively insensitive to the illumination wavelength [11] . We demonstrate this broadband feature by illuminating the HPP strips with visible and near-infrared light ( λ =633, 808 and 1,427 nm) and find that the vertical mode confinement remains essentially constant at about 50–60 nm ( Fig. 2c ). Since the chosen HPP strip height, H , is purposely kept constant through all experiments, a subtle mode height increase is expected for changing the illumination wavelength from visible to near infrared. The confinement of the mode width is also deep sub-wavelength with λ /12 and λ /7 for visible and near-infrared wavelengths, respectively ( Fig. 2d ). These remarkably small mode sizes are among the smallest for propagating electromagnetic waves demonstrated to date and consequently facilitate reduced waveguide cross-talk leading towards high data bandwidth densities ( Supplementary Fig. S3 ). Figure 2: HPP mode confinement. ( a ) Experimental field intensity (black dots) of the HPP mode compared with different tip-sample separations, t , from its exiting point. The optical mode height of FWHM z =53 nm is deep sub-wavelength for λ =633 nm, HPP strip dimensions H =230 nm, W =174 nm. Note, the NSOM operates in tapping-mode having an average separation of t =10 nm (black line), and the simulated mode profile ( t =2 and 5 nm, red dotted and black dashed line, respectively) at this distance agrees well with the NSOM result. ( b ) Summary of experimental HPP mode dimensions yielding the smallest measured mode area of 53×63 nm 2 , at λ =633 nm. The good agreement between experimental data (mode width and height, black squares and red triangles, respectively) and theoretical simulations (dashed lines, colours, respectively) confirms that the optical HPP mode is indeed squeezed into the low dielectric constant gap: the mode height is independent on the strip width (triangles), whereas the mode width is scaling with the strip width (squares). ( c , d ) Line scans of the mode height and width for wavelengths of the illumination beam of 633, 808 and 1,427 nm featuring broadband, deep sub-wavelength operation of HPP-based devices. The FWHM (solid line) are Gaussian fits to binned data, yielding measured mode areas of λ 2 /120, λ 2 /59 and λ 2 /157, which are deep sub-wavelength modes for all three wavelengths. As the strip height, H , is optimized for 633 nm, a slightly larger mode height for longer excitation wavelengths is expected. Full size image Propagation length In addition to providing strong optical confinement, another advantage of the HPP mode, over other non-resonant plasmonic schemes [9] , [10] , [22] , [23] , [24] , [25] , is reduced optical loss by allocating most of the optical energy in the dielectric gap instead of inside the metal. We have measured the transmission through HPP strips of varying length under white light illumination ( Fig. 3a ). The sub-wavelength-confined HPP mode propagates more than ten times its vacuum wavelength at visible wavelengths near 633 nm, which is more than six times further than plasmonic control strips consisting of a metal-semiconductor interface without the low-index gap region ( Fig. 3b ). The propagation length increases with the wavelength, and exceeds 20 times its vacuum wavelength at near infrared (−0.3 dB μm −1 ; inset Fig. 3 ), thus allowing for sufficiently long interaction lengths, which, combined with strong optical confinement, can create strong light-matter interaction effects for active photonic components [15] , [16] , [17] . 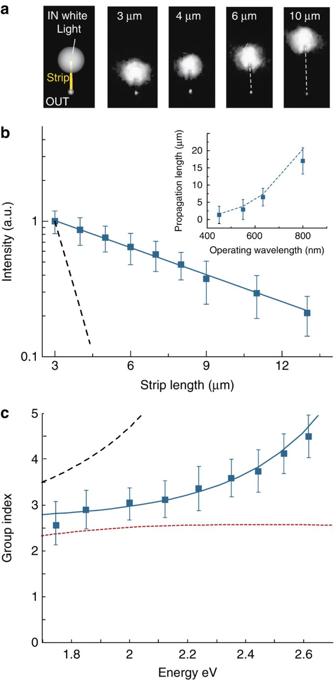Figure 3: HPP mode propagation length and mode speed. (a) Far field images of illuminated HPP strips showing incident white light reflected from the strip input and the corresponding emission from the distal strip output facet. The strip lengths,L, are indicated on top of each image and dashed lines guide the eye to the output signal. (b) The HPP mode offers propagation lengths of more than ten times its free-space wavelength atλ=633 nm (blue squares). Without the dielectric constant gap-layer (plasmonic control) the propagation length is only about 1 μm (black dashed line). Inset: the HPP mode's propagation length increases with its operating wavelength and exceeds 20 times its vacuum wavelength (0.3 dB μm−1) at near-infrared wavelength (λ=808 nm). The data (blue squares) are in good agreement with the expected trend from numerical calculations (blue dashed line; seeMethods). (c) HPP mode group index versus photon energy. Analysis of the HPP strip's transmission spectra, that is, Fabry–Perot interference for a range of strip lengths yields a dispersive group index of the HPP mode falling between the two extreme cases, that is, photonic (without metal, red dotted line) and plasmonic control (black dashed line) confirming the hybrid nature of the HPP mode. Figure 3: HPP mode propagation length and mode speed. ( a ) Far field images of illuminated HPP strips showing incident white light reflected from the strip input and the corresponding emission from the distal strip output facet. The strip lengths, L , are indicated on top of each image and dashed lines guide the eye to the output signal. ( b ) The HPP mode offers propagation lengths of more than ten times its free-space wavelength at λ =633 nm (blue squares). Without the dielectric constant gap-layer (plasmonic control) the propagation length is only about 1 μm (black dashed line). Inset: the HPP mode's propagation length increases with its operating wavelength and exceeds 20 times its vacuum wavelength (0.3 dB μm −1 ) at near-infrared wavelength ( λ =808 nm). The data (blue squares) are in good agreement with the expected trend from numerical calculations (blue dashed line; see Methods ). ( c ) HPP mode group index versus photon energy. Analysis of the HPP strip's transmission spectra, that is, Fabry–Perot interference for a range of strip lengths yields a dispersive group index of the HPP mode falling between the two extreme cases, that is, photonic (without metal, red dotted line) and plasmonic control (black dashed line) confirming the hybrid nature of the HPP mode. Full size image Mode group index interference measurements To gain full insight into the HPP mode physics, we also investigated the mode speed, namely the group index, n g . The abrupt change in the effective refractive index at the end of the HPP strip acts as a partial reflector for the HPP modes. The resulting optical cavity displays Fabry–Perot interference fringes, corresponding to longitudinal cavity modes. The group index can be determined from the spectral mode spacing, Δ λ =( λ 2 /2 n g L ), where L is the strip length, λ the wavelength, n g =n −d n /d λ the group index and n is the effective mode index. The increasing group index with photon energy confirms the dispersive, plasmonic mode character of the HPP mode, which manifests itself in the deep sub-wavelength confinement ( Fig. 3c ). In contrast, an effective mode group index close to one of the other surface plasmon polariton-based designs indicates that most of the field sits outside the metal, thus showing only weak optical confinement [23] . The dispersion of the HPP relation lies between the two extreme cases of gap width, h : namely, a semiconductor strip ( h →∞) and a semiconductor strip in direct contact with the silver film ( h →0). This demonstrates controlled hybridization of the modes of a semiconductor strip and a metal–dielectric interface. Plasmonic waveguides can be deployed in two distinct application areas: routing information passively [8] , [9] , [10] , [11] , [22] , [23] , [24] , [25] and actively altering optical signals [15] , [16] , [17] . For the latter, the optical confinement can strengthen light-matter interactions, thereby reducing the required devices size to utilize a certain effect (for example, a 2nd, 3rd order nonlinearity). The trade-off lies in enhancing such effect, that is, mode confinement, and incurring loss over the designed device length providing the effect. With this in mind, deep sub-wavelength metal optics hold promise to produce a significant nonlinear enhancement, while maintaining sufficient propagation distances leading to unprecedented footprint-performance functions. In conclusion, we directly demonstrated waveguiding of ultra-small propagating waves [11] at visible and near-infrared frequencies using NSOM imaging. We confirm the appropriate optical field hybridization between a surface plasmon and a dielectric mode by Fabry–Perot interference spectroscopy and find a dispersive group index as a result. This HPP concept has reduced ohmic losses offering reasonably long light-matter interaction lengths, potentially enabling compact and efficient nanoscale photonic components, as it elegantly interfaces plasmonics with semiconductors. This novel mode design holds a great potential for truly nanoscale photonic applications, such as intra-chip optical communication [19] , signal modulation [15] , [16] , [17] , nanoscale lasers [13] and biosensing [28] . Sample fabrication and experimental details Lithographically defined hybrid plasmon mode strips are prepared by evaporating a high-index semiconductor, ZnS, n =2.2 onto an Ag film separated by a thin, h =10 nm, MgF 2 film, both on a quartz substrate followed by lift off in acetone. The root-mean-square of the Ag film roughness is about 1.0–1.5 nm, measured using atomic force microscopy. The strip input was chosen to be tapered to act as an optical funnel to increase the signal strength and to reduce the impedance mismatch between free space and the HPP mode (inset Fig. 1b ). Focused ion beam milling creates the input and the 45° angled output port to enable the scanning NSOM tip to access the HPP mode's field profile. HPP strip illumination for the NSOM experiments is achieved by focusing a laser beam from the sample backside (quartz) with the following wavelengths: a He–Ne laser at λ =633 nm and two solid-state laser diodes at 808 and 1,427 nm wavelength, respectively ( Fig. 1a ). For the mode decay length and speed measurements a white light (Xe lamp, 150 W) illuminates the HPP strip in a reflection mode setup ( Supplementary Fig. S1b ). The signal to noise ratio was increased by placing an aperture in the secondary plane of the image, that is, over the end of the strip. The transmitted signal is then collected by an objective lens (×100, numerical aperture=0.9), sent to a spectrometer and recorded by an N 2 -cooled CCD camera. All measurements were carried out at room temperature. The mode's decay length is measured by the change in the absolute intensity with the variation of the strip length. The experimental results from Figure 3b are in good agreement with that obtained by simulation. Data from ref. 29 were used for the wavelength-dependent propagation length calculation showing good agreement with the experimental results ( Fig. 3b ). In an earlier work, we found that the permittivity values from Johnson and Christy [29] were overestimations by about 40% (ref. 30 ), which, together with additional scattering losses, could explain the small difference between experiment and simulation results. For the group index extraction from the measurement data, the Drude-model was used with the following parameters; the refractive indexes for air, zinc sulphide and magnesium floride were 1, 2.2 and 1.4, respectively; for silver we used ɛ Ag ( λ =600 nm)=−16.10–0.44 i (ref. 29 ). How to cite this article: Sorger, V. J. et al . Experimental demonstration of low-loss optical waveguiding at deep sub-wavelength scales. Nat. Commun. 2:331 doi: 10.1038/ncomms1315 (2011).